Legumain protease-activated TAT-liposome cargo for targeting tumours and their microenvironment Specific targeting and cellular internalization are key properties for carriers of antitumor therapeutic agents. Here, we develop a drug carrier through the attachment of substrate of endoprotease legumain, alanine–alanine–asparagine (AAN), to cell-penetrating peptides (TAT, trans-activating factor). The addition of the AAN moiety to the fourth lysine in the TAT creates a branched peptide moiety, which leads to a decrease in the transmembrane transport capacity of TAT by 72.65%. Legumain efficiently catalyses the release of TAT-liposome from the AAN-TAT-liposome and thereby recovers the penetrating capacity of TAT. Doxorubicin carried by the AAN-TAT-liposome led to an increase in the tumoricidal effect of doxorubicin and a reduction in its systemic adverse effects in comparison with doxorubicin carried by a control delivery system. Thus, the specific targeting and high efficiency of this delivery platform offers a novel approach to limit the toxicity of anticancer agents as well as increasing their efficacy in cancer therapy. Efficient delivery systems are an important prerequisite to the achievement of successful targeted anticancer agents [1] , [2] . Liposome-based nanoparticles have been used previously as drug carry systems because they can be readily modified and generally exhibit good compatibility towards a range of different therapeutic agents, including small molecules, proteins and even short interfering RNA [3] , [4] , [5] . Although a variety of different strategies have been proposed to improve the properties of drug-loaded liposomes, including efforts to prolong their circulation time, increase their internalization, and improve their target efficacy, research in these areas has so far been largely unsuccessful and the development of a multitask delivery platform is therefore still urgently required [6] . TAT peptide is one of the most frequently used cell-penetrating peptides (CPPs) and a powerful internalization moiety which has been widely used in the modification of drug delivery systems [7] . TAT peptide conjugation has been shown to enhance the cellular uptake of doxorubicin-loaded liposomes, as well as improving transfer across the blood brain barrier in in vitro models [8] . TAT-based modification through the formation of direct links to the liposome surface, however, can lead to endocytosis and a lack of cell-specificity, which in turn accelerates elimination through the mononuclear phagocyte system [9] . The combination of a cell-penetrating peptide with a targeting peptide conjugate has recently been reported as a potential strategy to achieve cell-type selective uptake of TAT modified liposomes [10] , [11] , [12] . In terms of improving the targeting efficacy of anticancer agents, trends in modifications have shifted from primarily attacking the tumour cells themselves to targeting specific areas at the tumour site. Recent studies also suggested that the tumour microenvironment plays a critical role in the initiation and progression of malignant carcinoma [13] , [14] . In fact, the design of carrier systems to specifically target the neovasculature of the tumour has been demonstrated as an effective strategy in cancer treatment. Several other reports also identified tumour-associated macrophages (TAMs) as promising therapeutic targets in a range of different tumour types. The targeted depletion of TAMs, using either a mini-gene vaccine or a doxorubicin-based drug has been shown to alleviate tumour growth and metastases in murine tumour models [15] , [16] , [17] , [18] . Legumain is a highly conserved lysosomal/vascuolar cysteine protease, which was originally identified in legumes [19] . Under physiological conditions, legumain is primarily expressed in kidney tubuli and contributes to renal tubular reabsorption [20] , [21] . Results of several studies have indicated that legumain expression is upregulated in a variety of different solid tumour types to a level that is positively correlated with the potential of malignancy [22] , [23] , [24] . As well as tumour cells themselves, several other cell types in the tumour-associated microenvironment have also been reported to express high levels of legumain, especially TAMs [14] , [16] . In addition, sites of legumain expression were shown to move from the cellular plasma to the cell surface on stress, such as hypoxia and starvation [25] . On the basis of these changes in its specific expression pattern, legumain represents a good candidate molecule for the design of an anticancer drug carrier. Several different delivery systems based on legumain have been created and used effectively as carriers for anticancer agents [16] , [25] , [26] . Here, we describe the construction of a novel liposome-based drug delivery platform via the incorporation of an internalizing TAT modification and legumain-based tumour targeting. This particular design strategy allowed for liposomal nanoparticles to remain stable until they were recognized and subsequently cleaved by active legumain at the tumour site. Following the release of this blocking moiety, TAT effectively enhances the internalization of liposomes to allow for cell-type selective uptake. Specific legumain expression patterns at the tumour sites Legumain expression levels were examined in microarrays of several different tumour tissues, including samples from 370 breast cancer patients, 121 lung cancer patients and 80 lymphoma patients. The results of this analysis were in agreement with those previously published in the literature, with legumain expression being highly upregulated in a diverse range of tumour tissue types ( Fig. 1a ). In contrast, legumain expression occurred randomly in the adjacent normal tissue. Furthermore, legumain expression levels appeared to be positively correlated with the clinical stages of the tissue microarrays of breast and lung cancer patients ( Fig. 1b,c ). No significant differences were found in the legumain expression levels between the three pathological grades ( Supplementary Fig. 1a ) or the primary tumour sites and metastatic loci ( Supplementary Fig. 1b ). We also determined legumain expression levels in the TAMs of human breast cancer tissue samples as well as primary tumour tissue samples taken from mouse 4T1 breast cancer models. The results of these analyses revealed that the positive staining of legumain overlaid well with positive staining of CD68 or F4/80, which are markers of macrophages ( Fig. 1d ). 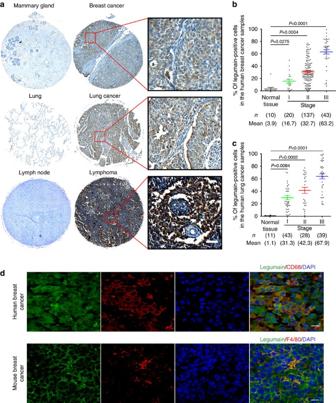Figure 1: Legumain expression profiles in tumours. Immunohistochemical staining was performed in a diverse range of tissue microarrays of tumours with the anti-legumain antibody. (a) Representative images of legumain expression in the human breast cancer microarrays (including 210 samples), lung cancer microarrays (including 121 samples), lymphoma microarrays (including 80 samples) and normal tissues adjacent to the tumour. Scale bar, 100 μm. The percentages of legumain positive cells per field were measured and the clinical stages identified by pathological diagnosis. The graphic represents the relationship between the percentage of legumain positive cells and the clinical stages of breast cancer (b) and lung cancer (c). Each point represents one sample and the middle line represents the mean value. Data are shown as the mean values±s.e.m. The number of samples and mean values of each group are listed below the x-axis. (P-value was determined by unpairedt-test). (d) Double stained sections of human and mouse breast cancers. Legumain is green and the CD68+or F4/80+macrophages are colored red. Scale bar, 10 μm. Figure 1: Legumain expression profiles in tumours. Immunohistochemical staining was performed in a diverse range of tissue microarrays of tumours with the anti-legumain antibody. ( a ) Representative images of legumain expression in the human breast cancer microarrays (including 210 samples), lung cancer microarrays (including 121 samples), lymphoma microarrays (including 80 samples) and normal tissues adjacent to the tumour. Scale bar, 100 μm. The percentages of legumain positive cells per field were measured and the clinical stages identified by pathological diagnosis. The graphic represents the relationship between the percentage of legumain positive cells and the clinical stages of breast cancer ( b ) and lung cancer ( c ). Each point represents one sample and the middle line represents the mean value. Data are shown as the mean values±s.e.m. The number of samples and mean values of each group are listed below the x-axis. ( P -value was determined by unpaired t -test). ( d ) Double stained sections of human and mouse breast cancers. Legumain is green and the CD68 + or F4/80 + macrophages are colored red. Scale bar, 10 μm. Full size image Construction and characteristics of the AAN-TAT-Lipo The polypeptide GGG-GRKK(AAN)RRQRRRQC was synthesized and linked to liposomal nanoparticles ( Fig. 2 ) to provide liposomal nanoparticles, which were modified with alanine–alanine–asparagines (AAN; protease substrate) and TAT, where the transmembrane transport capacity of TAT was blocked by AAN conjugated at the site of the fourth lysine. Analysis of the AAN-TAT-Lipo nanoparticles by transmission electron microscopy revealed that they had a uniform spherical shape with a diameter of 112.3±24.6 nm (mean±s.e.m., n =6), and dynamic light scattering analysis revealed that they were electrically neutral at pH 7.0 ( Supplementary Fig. 2 ). 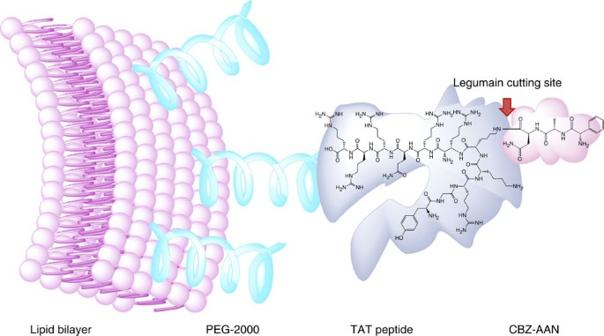Figure 2: Schematic diagram of AAN-TAT-Lipo nanoparticle structure and its legumain-cleavable site. The polypeptide GGG-GRKK(AAN)RRQRRRQC was linked to liposomal nanoparticles. Figure 2: Schematic diagram of AAN-TAT-Lipo nanoparticle structure and its legumain-cleavable site. The polypeptide GGG-GRKK(AAN)RRQRRRQC was linked to liposomal nanoparticles. Full size image Active legumain cleaves AAN from the AAN-TAT-Lipo The catalytic activity of legumain on the synthesized nanoparticles was measured. The lysates of the 4T1 cells overexpressing legumain or the CoCl 2 -stimulated 4T1 cells under hypoxic condition were used as sources of active legumain for our in vitro studies of legumain activity. A specific legumain inhibitor was used to validate the specificity of legumain activity. Increases in the active form of legumain in the lysates of each experimental group were compared with those of respective controls by western blot analysis ( Fig. 3a,b ). The higher ratio of active legumain to pro-legumain in the lysates of CoCl 2 -stimulated 4T1 cells suggested that more of the active legumain form was generated under CoCl 2 -stimulated hypoxic condition ( Fig. 3c ). The AAN-specific reorganization and enzymatic cleavage activities of the lysates of legumain overexpressing or CoCl 2 -stimulated 4T1 cells were confirmed using the commercial substrate Z-AAN-AMC at pH 6.0. The signal of the AMC molecule was used to represent the enzymatic activity of legumain ( Fig. 3d ). AAN cleavage activity in the lysate of legumain-overexpressing 4T1 cells was significantly suppressed in the presence of the legumain inhibitor ( Fig. 3e ). To test whether active legumain could cleave AAN from the AAN-TAT-Lipo nanoparticles, AAN was labelled with FITC and doxorubicin loaded into the nanoparticles to visualize AAN and liposome, respectively. Characteristic peaks were observed at 520 and 590 nm in the luminescence spectra of these materials, which represented FITC-AAN and TAT-Lipo-Dox, respectively ( Fig. 3f ). Our results revealed a decrease in the FITC characteristic peak at 520 nm after treatment with active purified legumain, the lysate of the legumain-overexpressing 4T1 cells, or the lysate of the CoCl 2 -stimulated 4T1 cells. Furthermore, the decrease in the FITC characteristic peak induced by active purified legumain could be antagonized by the legumain inhibitor ( Fig. 3g,h ). Accordingly, downregulation of legumain via lentivirus transfection in 4T1 or MDA-MB-231cells ( Supplementary Fig. 3a ) also significantly suppressed the AAN cleavage activity when compared with controls ( Supplementary Fig. 3b,c ). Furthermore, a decrease in the FITC characteristic peak induced by legumain in the lysates of MDA-MB-231 cells ( Supplementary Fig. 3d ) and 4T1 cells with or without CoCl 2 stimulation ( Supplementary Fig. 3e ), could be antagonized by silencing down legumain. 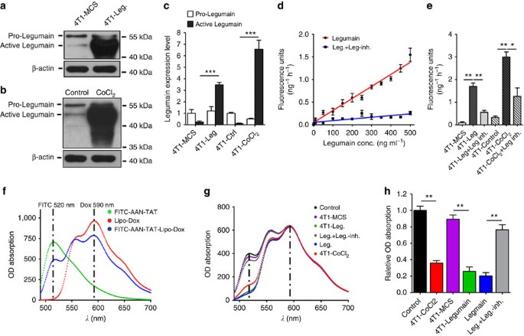Figure 3: Active legumain protease recognizes and cleaves AAN-TAT-Lipoin vitro. We established a stable 4T1 cell line overexpressing legumain by using a lentivirus infection system. Cell lysates were collected from the overexpressing legumain 4T1 cells and the control, together with the lysates of 4T1 cells treated with or without CoCl2for 24 h. (a) Western blot analysis of pro-legumain (about 56 kDa) and active legumain (about 46 kDa) in the lysates of the 4T1 cells overexpressing legumain or the control and (b) lysates of 4T1 cells treated with or without CoCl2(n=3). Quantification of the results from three independent experiments are shown inc. The values are shown as mean±s.e.m. (***P<0.001, determined by two-way analysis of variance). Activity and specificity properties of the endogenous legumain in the lysates were measured with Z-AAN-AMC. Purified mouse legumain and, legumain plus a legumain-specific inhibitor were separately incubated with the legumain substrate Z-AAN-AMC for 2 h. (d) Level of AMC release was recorded as OD value. The values are shown as mean±s.e.m. Lysates of the legumain-overexpressing 4T1 cells and the control, with or without the legumain-specific inhibitor, were incubated with Z-AAN-AMC (n=6). (e) Graphic bars represent the quantification of the AMC levels in the different groups. The values are shown as mean values±s.e.m. (*P<0.05, **P<0.01, determined by one-way analysis of variance). To visualize the legumain-mediated cleavage of AAN-TAT-Lipo particles, the AAN-TAT complex was labelled with FITC and resulting liposome was loaded with doxorubicin. FITC-labelled AAN-TAT-Lipo nanoparticles were also loaded with doxorubicin. Results of the spectral screening are shown inf. Two specific absorption peaks were observed at 520 and 590 nm. The FITC-labelled AAN-TAT-Lipo particles loaded with doxorubicin were separately incubated with lysates from the legumain-overexpressing 4T1 cells or control 4T1 cells, recombinant legumain protein or legumain plus legumain-specific inhibitor, and the lysates of the 4T1 cells following 24 h of CoCl2treatment. Results of spectral screening are shown ing. (h) Bar graphs represent the statistical results (n=3). The values shown represent the mean values±s.e.m (**P<0.01, determined by unpairedt-test). Figure 3: Active legumain protease recognizes and cleaves AAN-TAT-Lipo in vitro . We established a stable 4T1 cell line overexpressing legumain by using a lentivirus infection system. Cell lysates were collected from the overexpressing legumain 4T1 cells and the control, together with the lysates of 4T1 cells treated with or without CoCl 2 for 24 h. ( a ) Western blot analysis of pro-legumain (about 56 kDa) and active legumain (about 46 kDa) in the lysates of the 4T1 cells overexpressing legumain or the control and ( b ) lysates of 4T1 cells treated with or without CoCl 2 ( n =3). Quantification of the results from three independent experiments are shown in c . The values are shown as mean±s.e.m. (*** P <0.001, determined by two-way analysis of variance). Activity and specificity properties of the endogenous legumain in the lysates were measured with Z-AAN-AMC. Purified mouse legumain and, legumain plus a legumain-specific inhibitor were separately incubated with the legumain substrate Z-AAN-AMC for 2 h. ( d ) Level of AMC release was recorded as OD value. The values are shown as mean±s.e.m. Lysates of the legumain-overexpressing 4T1 cells and the control, with or without the legumain-specific inhibitor, were incubated with Z-AAN-AMC ( n =6). ( e ) Graphic bars represent the quantification of the AMC levels in the different groups. The values are shown as mean values±s.e.m. (* P <0.05, ** P <0.01, determined by one-way analysis of variance). To visualize the legumain-mediated cleavage of AAN-TAT-Lipo particles, the AAN-TAT complex was labelled with FITC and resulting liposome was loaded with doxorubicin. FITC-labelled AAN-TAT-Lipo nanoparticles were also loaded with doxorubicin. Results of the spectral screening are shown in f . Two specific absorption peaks were observed at 520 and 590 nm. The FITC-labelled AAN-TAT-Lipo particles loaded with doxorubicin were separately incubated with lysates from the legumain-overexpressing 4T1 cells or control 4T1 cells, recombinant legumain protein or legumain plus legumain-specific inhibitor, and the lysates of the 4T1 cells following 24 h of CoCl 2 treatment. Results of spectral screening are shown in g . ( h ) Bar graphs represent the statistical results ( n =3). The values shown represent the mean values±s.e.m (** P <0.01, determined by unpaired t -test). Full size image Characteristics of transmembrane activity of AAN-TAT-Lipo We proceeded to investigate the in vitro transmembrane capacity of AAN-TAT-Lipo nanoparticles carrying doxorubicin with or without the removal of AAN. Through visualization of doxorubicin (nanoparticles) and β-actin (cell outline), our data demonstrated the transmembrane capability of liposomal nanoparticles to be increased significantly following their modification with TAT. This was documented by the internalization of AAN-TAT-Lipo nanoparticles being reduced significantly when compared with TAT-Lipo. However, treatment with CoCl 2 effectively recovered the internalization of the AAN-TAT-Lipo nanoparticles in cultured 4T1 mouse breast cancer cells ( Fig. 4a,b ). To evaluate the transmembrane capacity of AAN-TAT-Lipo carrying biomacromolecules, we also entrapped the enhanced green fluorescent protein (EGFP) plasmid in liposomal nanoparticles and then added them to the culture medium of 4T1 cells. Flow cytometry of EGFP was used to analyse internalization and activity of the EGFP plasmid. Results of this analysis suggested that the percentage of EGFP positive cells was markedly reduced from 77.5% in the TAT-Lipo-EGFP group to 27.4% in AAN-TAT-Lipo-EGFP group. Interestingly, the percentage of EGFP positive cells in the AAN-TAT-Lipo-EGFP group was recovered up to 63.5% following CoCl 2 treatment in the 4T1 cells ( Supplementary Fig. 4a,b ). 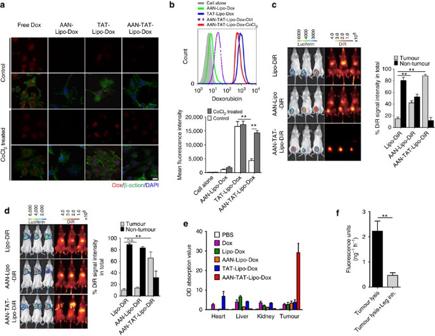Figure 4: AAN-TAT-Lipo enhances internalization of doxorubicin into CoCl2-stimulated 4T1 cells and its accumulation at the tumour site in an orthotopic mouse cancer model. Doxorubicin (1 nM) as well as an equivalent amount of doxorubicin loaded in different carriers was added to the culture medium of 4T1 cells treated with or without CoCl2. Immunofluorescence with an antibody against β-actin was used to visualize the region of cellular plasma. (a) Representative confocal microscopy images of the 4T1 cells. Scale bars, 5 μm. (b) Intensity of the doxorubicin fluorescence analysed by fluorescence-activated cell sorting. The values shown represent the mean±s.e.m. (n=3). (**P<0.01, determined by two-way analysis of variance). Mouse xenograft model of breast cancer and lung cancer was established via the orthotopic implantation of luciferase-expressing MDA-MB-231 cells or luciferase-expressing A549 cells, seperately. AAN-TAT-Lipo, AAN-Lipo or liposome alone were administrated intravenously when the tumour size reached approximately 500 mm3. To trace the particlesin vivo,the nanoparticles were all labelled with the near-infrared fluorescence probe DiR (n=3). (c,d) Bioluminescence images of the mice on administration of the luciferin substrate and images of the near-infrared fluorescence. Bar plot shows the distribution of DiR signal intensity at tumour sites and in liver regions. The values shown represent the mean±s.e.m. (**P<0.01, determined by two-way analysis of variance). In the MDA-MB-231 breast cancer mouse model, the tumour-bearing mice were given an equivalent amount of doxorubicin loaded into different carriers, respectively. The mice were killed 24 h later (n=8). (e) Bar plots represent concentrations of doxorubicin in different tissues. The values shown represent the mean values±s.e.m. Tumour lysates were prepared from the tumour tissues of the MDA-MB-231 mouse model and then incubated with legumain substrate Z-AAN-AMC for 1 h with or without the legumain inhibitor. (f) Results of the legumain activity assay. The values shown represent the mean±s.e.m. (n=3, **P<0.01, determined by Student’st-test). Figure 4: AAN-TAT-Lipo enhances internalization of doxorubicin into CoCl 2 -stimulated 4T1 cells and its accumulation at the tumour site in an orthotopic mouse cancer model. Doxorubicin (1 nM) as well as an equivalent amount of doxorubicin loaded in different carriers was added to the culture medium of 4T1 cells treated with or without CoCl 2 . Immunofluorescence with an antibody against β-actin was used to visualize the region of cellular plasma. ( a ) Representative confocal microscopy images of the 4T1 cells. Scale bars, 5 μm. ( b ) Intensity of the doxorubicin fluorescence analysed by fluorescence-activated cell sorting. The values shown represent the mean±s.e.m. ( n =3). (** P <0.01, determined by two-way analysis of variance). Mouse xenograft model of breast cancer and lung cancer was established via the orthotopic implantation of luciferase-expressing MDA-MB-231 cells or luciferase-expressing A549 cells, seperately. AAN-TAT-Lipo, AAN-Lipo or liposome alone were administrated intravenously when the tumour size reached approximately 500 mm 3 . To trace the particles in vivo, the nanoparticles were all labelled with the near-infrared fluorescence probe DiR ( n =3). ( c,d ) Bioluminescence images of the mice on administration of the luciferin substrate and images of the near-infrared fluorescence. Bar plot shows the distribution of DiR signal intensity at tumour sites and in liver regions. The values shown represent the mean±s.e.m. (** P <0.01, determined by two-way analysis of variance). In the MDA-MB-231 breast cancer mouse model, the tumour-bearing mice were given an equivalent amount of doxorubicin loaded into different carriers, respectively. The mice were killed 24 h later ( n =8). ( e ) Bar plots represent concentrations of doxorubicin in different tissues. The values shown represent the mean values±s.e.m. Tumour lysates were prepared from the tumour tissues of the MDA-MB-231 mouse model and then incubated with legumain substrate Z-AAN-AMC for 1 h with or without the legumain inhibitor. ( f ) Results of the legumain activity assay. The values shown represent the mean±s.e.m. ( n =3, ** P <0.01, determined by Student’s t -test). Full size image AAN-TAT-Lipo-Dox nanoparticles increased targeted enrichment Targeting efficiency of AAN-TAT-Lipo nanoparticles was also tested in vivo . Thus, DiR was manipulated to trace liposomal nanoparticles in an established xenograft mouse model of breast cancer with luciferase-expressing MDA-MB-231 breast cancer cells, as well as in a mouse model of lung cancer with luciferase-expressing A549 lung cancer cells. Equivalent volumes of DiR-labelled liposomes or AAN-lipo or AAN-TAT-Lipo nanoparticles were administrated to tumour-bearing mice via tail vein injection. Results revealed an enrichment in AAN-TAT-lipo nanoparticles at the tumour site, whereas the majority of the liposomal or AAN-Lipo nanoparticles were distributed in liver and spleen ( Fig. 4c,d ). Similar results were obtained in the animal model established with luciferase-expressing 4T1 cells ( Supplementary Fig. 5 ). To further evaluate the tissue distribution of the drug carried within the AAN-TAT-Lipo nanoparticles, we performed another set of in vivo experiments with nanoparticles carrying doxorubicin. Analysis of doxorubicin concentration in different tissues showed that this drug was efficiently enriched in tumour tissue of the AAN-TAT-Lipo group ( Fig. 4e ). Fluorescence analysis allowed for location of the doxorubicin to be visualized at different tissue regions ( Supplementary Fig. 6 ). Results of this analysis also suggested that the AAN-TAT-Lipo nanoparticles produced better tumour targeted effects when compared with liposomal nanoparticles. Interestingly, AAN cleavage by tumour tissue homogenates isolated from a xenograft mouse model of breast cancer was significantly suppressed in the presence of a legumain inhibitor ( Fig. 4f ). Together, these data underlined the tumour-targeting effect of AAN-TAT-Lipo in vivo. AAN-TAT-Lipo nanoparticles selectively targeted M2 macrophages It has been widely reported that M2-polarized macrophages account for the majority of TAMs; meanwhile, legumain expression is upregulated in M2 macrophages. Our data indicate that M2 polarization selectively induced by interleukin-4 (IL-4) promoted internalization of AAN-TAT-Lipo-Dox in macrophages ( Fig. 5a–c ), as well as increased the degree of macrophages killing by doxorubicin in vitro ( Fig. 5d ). In vivo , our data also demonstrated the targeted depletion of M2-polarized macrophages in the AAN-TAT-Lipo-Dox group when compared with other groups ( Supplementary Fig. 7 ). 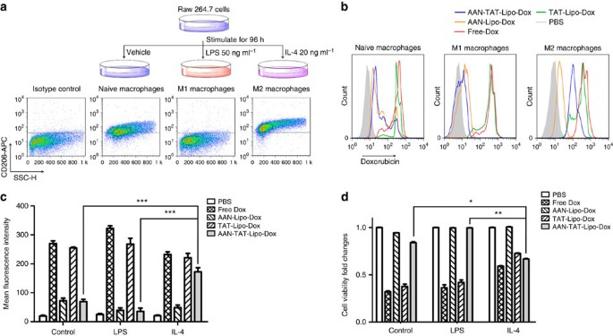Figure 5: AAN-TAT-Lipo selectively targets M2-polarized macrophagesin vitro. M1 or M2 polarization was induced in cultured RAW 264.7 cell by lipopolysaccharide or IL-4 separately for 96 h. Then, cells were treated with 1 nM doxorubicin or an equivalent amount of doxorubicin loaded into AAN-TAT-Lipo, AAN-Lipo or TAT-Lipo. Fluorescence-activated cell sorting analysis was performed 2 h after treatment of nanoparticles. (a) Upper panel illustrates the different subtypes of macrophages polarization. Representative flow cytometry plots of the CD206 positive cells are presented in the lower panel. (b) Representative fluorescence intensities of doxorubicin analyseds by FACS. Statistical results for the fluorescence intensities are shown inc. Cell viability assay was performed 24 h after the treatment of nanoparticles. Data represent mean values±s.e.m. (***P<0.001, determined by two-way analysis of variance). (d) Bar graphs represent results of cell viability assays from three independent experiments. Data shown here represent mean values±s.e.m. (*P<0.05, **P<0.01, determined by two-way analysis of variance). Figure 5: AAN-TAT-Lipo selectively targets M2-polarized macrophages in vitro . M1 or M2 polarization was induced in cultured RAW 264.7 cell by lipopolysaccharide or IL-4 separately for 96 h. Then, cells were treated with 1 nM doxorubicin or an equivalent amount of doxorubicin loaded into AAN-TAT-Lipo, AAN-Lipo or TAT-Lipo. Fluorescence-activated cell sorting analysis was performed 2 h after treatment of nanoparticles. ( a ) Upper panel illustrates the different subtypes of macrophages polarization. Representative flow cytometry plots of the CD206 positive cells are presented in the lower panel. ( b ) Representative fluorescence intensities of doxorubicin analyseds by FACS. Statistical results for the fluorescence intensities are shown in c . Cell viability assay was performed 24 h after the treatment of nanoparticles. Data represent mean values±s.e.m. (*** P <0.001, determined by two-way analysis of variance). ( d ) Bar graphs represent results of cell viability assays from three independent experiments. Data shown here represent mean values±s.e.m. (* P <0.05, ** P <0.01, determined by two-way analysis of variance). Full size image AAN-TAT-Lipo-Dox nanoparticles increase the tumoricidal effect The ability of a drug loaded into AAN-TAT-Lipo to exert a tumoricidal effect in a robust animal tumour model will determine its success as an effective delivery system. To evaluate the therapeutic efficacy of doxorubicin carried by the AAN-TAT-Lipo carrier system, a mouse orthotopic luciferase-expressing 4T1 breast cancer model was treated with AAN-TAT-Lipo-Dox as well as several other control nanoparticle systems ( Fig. 6a ). Results of bioluminescence signal capture and tumour growth measurements revealed that tumour growth was significantly slower in the AAN-TAT-Lipo-Dox administration group than in the other treatment groups ( Fig. 6b,c ). Furthermore, AAN-TAT-Lipo-Dox significantly prolonged survival periods of tumour-bearing mice ( Fig. 6d ). When loaded with an equivalent dose of the drug, results of terminal deoxynucleotidyl transferase dutp nick end labeling staining indicated a 65.4% apoptotic rate at the tumour site in the AAN-TAT-Lipo-Dox treatment group as compared to much lower apoptotic rates of only 1.2, 5.7 and 16.9% in the free Dox, AAN-Lipo-Dox and TAT-Lipo-Dox treatment groups, respectively ( Fig. 6e,f ). Furthermore, rates of apoptosis in heart, liver and kidney were reduced significantly in the AAN-TAT-Lipo-Dox treatment group when compared with any of the other treatment groups. These severe adverse effects could explain the similar survival periods observed in the phosphate-buffered saline (PBS), free Dox, AAN-Lipo-Dox and TAT-Lipo-Dox experimental groups, although the rate of tumour growth in the free Dox, AAN-Lipo-Dox and TAT-Lipo-Dox groups was much slower than that observed in the PBS control group ( Fig. 6c ). Taken together, these results demonstrate that AAN-TAT-Lipo nanoparticles significantly enhanced tumour-targeting efficacy of doxorubicin while reducing its systemic toxicity. 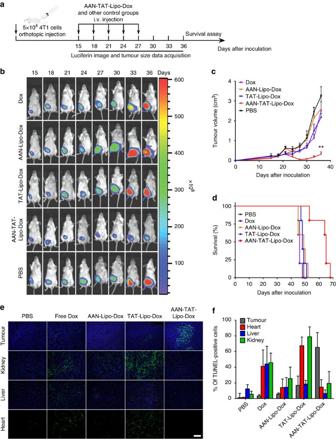Figure 6: AAN-TAT-Lipo increases accumulation at tumour sites and tumoricidal effects of doxorubicin in orthotopic 4T1 breast cancer models. A mouse model was established for breast cancer via the orthotopic implantation of 4T1 cells overexpressing luciferase. Forty mice were randomly divided into five groups and treated with AAN-TAT-Lipo-Dox or controls (n=8) as follows, AAN-Lipo-Dox, TAT-Lipo-Dox, AAN-TAT-Lipo-Dox, doxorubicin alone and PBS. (a) Illustration of the experimental design. (b) Representative bioluminescence images of mice following the administration of luciferin substrate. Images were taken at different time points after injection of tumour cells. Statistical results concerning tumour size are shown in (c). Data are presented as the mean values±s.e.m. (**P<0.01, determined by two-way analysis of variance). (d) Kaplan–Meier survival curve for mice bearing 4T1 tumours in different treatment groups. These survival data were based on the primary tumour diameter (>1.8 cm) and humane endpoints. (e) Terminal deoxynucleotidyl transferase dutp nick end labeling (TUNEL) staining was used to evaluate levels of apoptosis in the 4T1 tumours, as well as kidney, liver and heart tissues. Scale bar, 100 μm. The statistical results of the TUNEL staining are shown in (f). Data shown represent the mean values±s.e.m. Figure 6: AAN-TAT-Lipo increases accumulation at tumour sites and tumoricidal effects of doxorubicin in orthotopic 4T1 breast cancer models. A mouse model was established for breast cancer via the orthotopic implantation of 4T1 cells overexpressing luciferase. Forty mice were randomly divided into five groups and treated with AAN-TAT-Lipo-Dox or controls ( n =8) as follows, AAN-Lipo-Dox, TAT-Lipo-Dox, AAN-TAT-Lipo-Dox, doxorubicin alone and PBS. ( a ) Illustration of the experimental design. ( b ) Representative bioluminescence images of mice following the administration of luciferin substrate. Images were taken at different time points after injection of tumour cells. Statistical results concerning tumour size are shown in ( c ). Data are presented as the mean values±s.e.m. (** P <0.01, determined by two-way analysis of variance). ( d ) Kaplan–Meier survival curve for mice bearing 4T1 tumours in different treatment groups. These survival data were based on the primary tumour diameter (>1.8 cm) and humane endpoints. ( e ) Terminal deoxynucleotidyl transferase dutp nick end labeling (TUNEL) staining was used to evaluate levels of apoptosis in the 4T1 tumours, as well as kidney, liver and heart tissues. Scale bar, 100 μm. The statistical results of the TUNEL staining are shown in ( f ). Data shown represent the mean values±s.e.m. Full size image In this study, we initially evaluated legumain expression patterns in a variety of different human tumour tissue types. On the basis of its characteristic expression pattern in tumour tissues, legumain has been used extensively in the development of methods for the diagnosis of cancer as well as for development of novel strategies in treatment of cancer [23] , [26] , [27] . One of the most interesting ways in which legumain has been applied to the development of novel anticancer agents is in the design of antitumor prodrug platforms that specifically require asparagine at the P1 site of their substrate [28] . In fact, a prototype prodrug synthesized by the addition of doxorubicin to a legumain-specific substrate peptide through a peptide bond markedly reduced the toxicity of doxorubicin and increased its tumoricidal activity [29] . Another synthesized legumain-cleavable prodrug which was reported in the literature is carbobenzyloxy–alanine–alanine–asparagine–ethylenediamine–etoposide, which could be cleaved by either recombinant human legumain or ectopic overexpressed legumain in cultured tumour cells [30] . Despite these successes, there are several disadvantages associated with the direct linkage of an active drug to a protease substrate. For example, strategies of this type require specific models of design and synthesis for each drug because the formation of direct links to different drugs could be dependent on size, electronic characteristics and chemical constitution of the drug. With this in mind, we decided to use the specific substrate structure of legumain to modify liposomal nanoparticles and design a universal drug carrier platform for use in cancer therapy. Liposomal nanoparticles have emerged as optimal drug carriers because of their high efficacy, pronounced drug encapsulation ability and long circulation time in vivo [4] . Furthermore, the use of liposomal nanoparticles has been shown to have no discernible impact on the characteristics of the entrapped drug [31] . Previous studies in this area have indicated that the trans-activating factor (TAT) could promote the cell internalization capability of liposomal nanoparticles [32] , [33] . Notably, the beneficial effect of TAT penetration is mainly dependent on the fourth lysine residue of the TAT amino acid sequence. The mutation of this particular residue reduces the activity of TAT towards transmembrane transport by 70% [34] . Furthermore, lysine is the only natural amino acid bearing an amine moiety as its side chain. On the basis of these characteristics, the decision was taken to use a conjugate of the legumain substrate to TAT at the fourth lysine residue. It was envisaged that this design would make it possible to block the transmembrane activity of TAT before release of the legumain substrate. Our results showed that the addition of the AAN moiety to the fourth lysine residue in TAT decreased its transmembrane transport capacity by 72.65% in vitro . Therefore, active legumain could be used to effectively recover the internalization capacity of TAT. The biodistribution of empty or doxorubicin-loaded AAN-TAT-lipo nanoparticles was evaluated in vivo by detecting the fluorescence signals from labelled DiR and loaded doxorubicin. DiR tracing showed that AAN-TAT modification effectively eliminated any non-specific distribution and further improved the tumour-targeting efficiency when compared with the AAN-lipo and liposome groups. Analysis of the doxorubicin-loaded liposomal nanoparticles provided more detailed distribution data. Thus, the level of doxorubicin enrichment at the tumour site was significantly higher in the AAN-TAT-lipo group than in the control group. Interestingly, renal distribution of doxorubicin loaded with AAN-TAN-lipo nanoparticles was low. This result seems somewhat at odds with the observation that kidney is the major site of legumain expression under standard physiological conditions. However, we speculate the reason for this is due to the legumain expression in kidney to be at the renal tubular site. As we know, substances in circulation cannot reach the tubule until they are filtered by the glomerular filtration barrier. It is estimated that the mean diameter of the glomerular filtration barrier is around 40–60 nm. Therefore, the size of nanoparticles leads to their separation from the renal tubuli. In addition, legumain expression at the tubular sites is located in the lysosomes within the cytoplasm thus further hindering reorganization and digestion of nanoparticles. Upregulated legumain expression was observed in tumour cells as well as TAMs. Our data demonstrated that M2 polarization of macrophages when stimulated by IL-4, promotes uptake of AAN-TAT-Lipo-Dox in macrophages and increases the degree of macrophage killing by doxorubicin. Thus, this suggests that nanoparticles target not only tumour cells, but also the tumour microenvironment. Although thorough evaluation on the systemic toxicity in response to the target depletion of M2 macrophages is worthy, this dual-targeting characteristic of AAN-TAT-nanoparticles sheds light onto the therapeutic efficacy of this antitumor strategy, considering the important role of the tumour microenvironment in potentializing the malignancy of tumours. Taken together, our data demonstrated that AAN-TAT-Lipo cargo blocks TAT peptide activation with a legumain-specific substrate before the reorganization of the AAN by legumain at the tumour site. Once legumain has acted, the catalytic effect of AAN recovers the internalization efficacy of TAT. In conclusion, we believe that this novel drug delivery system could be used to achieve improved tumour targeting and prointernalization. Furthermore, this cargo is multifunctional in terms of its high compatibility with small molecules, short interfering RNA and proteins. This system could therefore be used to optimize antitumor therapeutic strategies and improve the prognosis of tumour patients. Immunohistochemistry and tissue microarray Legumain expression was detected in high-density tissue microarrays of breast cancer, lung cancer and lymphoma samples (Alenabio Co., Ltd, Xi’an, China). All human tissues are collected under institutional review board- and HIPPA-approved protocols. All samples have been tested negative for HIV and Hepatitis B or their counterparts in animals, and approved for commercial product development. For immunohistochemistry, paraffin sections were incubated overnight at 4 °C with the primary antibody after dewaxing and hydration. Antibody against legumain was used at 1:100 dilution (Santa Cruz Biotechnology, Inc., Santa Cruz, CA). Slides were then incubated with a biotinylated secondary antibody for 1.5 h before being exposed to a streptavidin–peroxidase complex for 0.5 h. Following visualizing with diaminobenzidine and counter-staining with hematoxylin, slides were dehydrated and mounted with neural resin. Legumain expression was quantified by counting the percentage of legumain positive cells in a microscopic field. Information pertaining to the tumour stages was provided by the supplier of the tissue microarrays. Immunofluorescence staining Human breast tumour tissues and tumour samples from the breast cancer mouse models were fast frozen after embedding with optimal cutting temperature compound. Slides of 5 μm in thickness were fixed with cold methanol at –20 °C for 20 min and then blocked in 2% bovine serum albumin for 1 h. Slides were then incubated with antibodies overnight at 4 °C. An antibody against legumain, F4/80 (Santa Cruz) or CD68 (DakoCytomation, Carpinteria, CA, USA), was used and subsequently incubated with an Alexa 488-labelled secondary antibody (Invitrogen, Carlsbad, CA, USA) and an Alexa 594-labelled secondary antibody (Invitrogen) for 1 h. For nuclear staining, cells were stained with 4′,6-diamidino-2-phenylindole. For immunofluorescence staining of cultured cells, they were fixed with 4% paraformaldehyde, and then incubated with anti-mouse β-actin antibody. 4′,6-diamidino-2-phenylindole was used for counter-staining of the nucleus. The tissue stained sections were mounted in Vectashield mounting medium (Vector Lab, Burlingame, CA, USA). Photographs were taken with a TCS-SP5 fluorescence confocal microscope (Leica Microsystems, Mannheim, Germany). Cell lines and reagents 4T1 murine breast cancer cells, A549 human lung cancer cells, MDA-MB-231 human breast cancer cells and murine macrophage RAW 264.7 were obtained from the American Type Culture Collection (Manassas, VA, USA). 4T1 and RAW 264.7 cells were cultured in RPMI-1640 medium, whereas A549 and MDA-MB-231 cells were cultured in Dulbecco’s Modified Eagle’s medium supplemented with 10% fetal bovine serum and 1% NEAA (Invitrogen). For establishing stable legumain-expressing and luciferase-expressing cell lines, 4T1 cells, MDA-MB-231 cells or A549 cells were infected with pLV-EF1α-Legumain-IRES-Bsd plasmid or pLV-EF1α-Luciferase-IRES-Bsd using a lentivirus transfection system (Biosettia, San Diego, CA, USA). The lentivirus production and infection steps were conducted in accordance with the manufacturer’s protocol and positive cells were selected using Blasticidin S at a concentration of 10 μg ml −1 (ref. 35 ). Cell lysates and conditioned medium were tested for legumain expression by western blot analysis. To stimulate hypoxia, cobalt chloride (CoCl 2 ), 100 mM CoCl 2 was added to 4T1 cells in the absence or presence of 100 nM of a legumain inhibitor, and the resulting mixture incubated for 12 h at 37 °C [36] . Free doxorubicin (1 nM) or an equivalent amount of doxorubicin loaded into AAN-TAT-Lipo or some other control nanoparticles were added to the culture medium. Cells were then collected for analysis by flow cytometry or immunofluorescence staining. To stimulate M1 or M2 polarization in macrophages, 50 ng ml −1 lipopolysaccharide (Sigma-Aldrich, St Louis, MO) or 20 ng ml −1 mouse interleukin 4 (IL-4; R&D, Minneapolis, MN) were added to the Raw 264.7 cells and the cells incubated for 96 h at 37 °C. Recombinant mouse legumain was purchased from Sino Biological Inc. (Beijing, China). The legumain substrate was purchased from AnaSpec Biological Inc (Fremont, CA, USA). Synthetic legumain inhibitor RR-11a [37] , [38] was synthesized by Wuxi Apptec Inc. (Beijing, China). The legumain-specific substrate Ala–Ala–Asn (AAN), TAT, the AAN-TAT conjugate at the fourth lysine of the TAT sequence and the FITC-labelled AAN-TAT were custom synthesized by Ziyu peptide Inc (Shanghai, China). DiR dye was purchased from Invitrogen. Flow cytometry assay 4T1 cells were seeded in six-well cell culture plates at 0.3 × 10 6 cells per well with or without hypoxia induction by CoCl 2 for 24 h, and the cells were then treated with 1 nM doxorubicin or an equivalent amount of doxorubicin loaded in AAN-TAT-Lipo, AAN-Lipo or TAT-Lipo. After 1 h of treatment, each well was washed with PBS and the cells were dissociated with 0.25% trypsin and resuspended at 10 6 cells ml −1 in Hanks Buffered Salt Saline supplemented with 2% FBS and 1% HEPES. The resulting suspension was immediately analysed using a digital BD Caliber flow cytometer (BD Biosciences, San Jose, CA, USA) with an excitation wavelength of 550 nm and 30,000 events being collected per sample. Data were analysed using FlowJo software (Tree Star, Inc, Ashland, OR, USA). For the experiment with macrophages, the polarized Raw 264.7 cells were seeded in six-well plates at 0.3 × 10 6 cells per well, and cells were then treated as described above, except the resulting suspension was stained with CD206-APC antibody (Santa Cruz Biotechnology) before being analysed by flow cytometry. Cell viability assay Polarized Raw 264.7 cells were seeded in 96-well plates at 2,000 cells per well, and the cells were then treated with 1 nM doxorubicin or an equivalent amount of doxorubicin loaded to AAN-TAT-Lipo, AAN-Lipo or TAT-Lipo. After treatment of doxorubicin, cell viability assay was performed according to the manufacturer’s protocol (Cell Counting Kit-8, Dojindo Laboratories, Kumamoto, Japan). Preparation and characterization of nanoparticles To prepare the AAN-TAT-Lipo nanoparticles, we initially dissolved the phospholipids (Avanti Polar Lipids Inc, Alabaster, AL, USA) in chloroform, AAN-TAT peptide was then conjugated to 1,2-dioleoyl- sn -glycero-3-phosphoethanolamine (DOPE) according to the procedure described below. The amino-terminal of the AAN-TAT peptide was converted to the NHS ester. To this end, 1:1 (mol/mol) mixture of DOPE and EDC was mixed with MES buffer at pH 5.0. AAN-TAT-NHS and DOPE were then mixed with EDC at a molar ratio of 1:1, and the pH of the mixture adjusted pH 9.0 for the conjugation process. The AAN-TAT-DOPE peptide was purified on a PD-10 column, and the resulting compound combined with 1,2-dioleoyl- sn -glycero-3-phosphocholine, DOPE, cholesterol and 1,2-dioleoyl- sn -glycero-3-phospho-ethanolamine- N -[methoxy(polyethylene glycol)-2000], DOPE-PEG2000 at a molar ratio of 1.1:6.7:6.7:2.2:1 [25] . Doxorubicin was loaded into the nanoparticles according to a modified version of a previously published procedure [39] . Briefly, the lipid film was rehydrated in 1 ml sterile ammonium phosphate buffer (300 mM, pH 7.4) with agitation for a minimum of 1 h. The material was then sonicated to produce 100-nm-scale nanoparticles. The exterior ammonium phosphate buffer was exchanged with PBS (pH 7.4) by gel-filtration chromatography over a PD-10 column (GE Healthcare, Buckinghamshire, UK). Ten micromoles doxorubicin was then added to the lipid film at a volume ratio of 1:100, and the resulting mixture incubated overnight at room temperature. The nanoparticles incorporated with doxorubicin were purified by gel-filtration chromatography over a PD-10 column using PBS buffer (pH 7.4) as the eluent. To prepare the pEGFP loaded nanoparticles, AAN-TAT-DOPE, 1,2-dioleoyl- sn -glycero-3-phosphocholine, DOPE, N -[1-(2,3-Dioleoyloxy)propyl]- N,N,N -trimethyl ammonium chloride (DOTAP), cholesterol and DOPE-PEG2000 were mixed at molar ratios of 1.1:6.7:6.7:2:2.2:0.5, respectively. The formulated nanoparticles were mixed with pEGFP plasmids at DOTAP and DNA molar ratios of 1:4 for 12 h at room temperature. To prepare the DiR-labelled nanoparticles, the AAN-TAT-Lipo or other nanoparticles were mixed with 10 μM dimethyl sulfoxide dissolved DiR at a volume ratio of 100:1, and the resulting mixture incubated at 37 °C for 2 h. The DiR-labelled nanoparticles were purified over a PD-10 column using PBS buffer (pH 7.4) as an eluent. The morphological characteristics of the nanoparticles were examined with a Philips T20ST transmission electron microscope (Amsterdam, Netherlands). An acceleration voltage of 200 kV was used for the transmission electron microscope analysis. The size and zeta potentials of the nanoparticles were measured with a ZetaPALS/90plus zeta potential analyzer (Brookhaven Instruments Corp, Holtsville, NY, USA). Western blot assay Confluent cells were collected with PBS for the western blot assay. Cells were centrifuged at 3,000 g for 5 min at 4 °C, and the resulting pellets resuspended in RIPA buffer. Protein concentration was then tested using a BCA kit. The cell lysates were boiled two times in sample buffer and loaded onto a 10% polyacrylamide gel. Proteins were then transferred onto a nitrocellulose membrane, which was subsequently incubated overnight at 4 °C with a primary antibody against legumain (1:1,000; sc-67163, Santa Cruz) before being blocked with 5% non-fat milk for 1 h. The membranes were then washed three times with tris-buffered saline and tween 20 and incubated with a horse-radish peroxidase-labelled secondary antibody for 1 h. The membranes were then washed three times with tris-buffered saline and tween 20 and incubated with an ECL kit before being exposed to film and developed. Blots probed with antibody against β-actin (1:5,000; Santa Cruz) were used to confirm equal loading. Full-length images of all immunoblots are shown in Supplementary Fig. 8 . Activity assay of legumain The commercial legumain substrate Z–Ala–Ala–Asn–AMC was used to evaluate the activation of legumain by comparing the AMC signals in the samples [40] . Before all of the activity assays, recombinant mouse legumain standard was activated by incubation at a concentration of 100 μg ml −1 in a mixture of 50 mM NaOAc and 0.1 M NaCl at pH 4.0 for 2 h at 37 °C. The specific activity of the legumain standard was diluted from 0 to 5 μg ml −1 and measured by using 100 μM of the commercial legumain substrate Z–Ala–Ala–Asn–AMC [41] . Cleavage of Z–Ala–Ala–Asn–AMC was measured at excitation and emission wavelengths of 353 and 442 nm, respectively, in a fluorescence plate reader (Gemini EM, Berkshire, UK). Ten microlitre samples of cell lysates or tumour tissue homogenates were placed in a 96-well plate and treated with 190 μl of a solution of Z–Ala–Ala–Asn–AMC in assay buffer to give a final substrate concentration of 10 μM. The plates were then incubated at 37 °C for 2 h and fluorescence levels of the released AMC were measured at excitation and emission wavelengths of 353 and 442 nm, respectively. Legumain-specific peptide Ala–Ala–Asn cleavage assay To validate the recognition and cleavage of AAN in the AAN-TAT-Lipo nanoparticle with active legumain, we constructed an FITC-labelled AAN peptide and loaded doxorubicin into the FITC-labelled AAN-TAT-Lipo nanoparticles. The cell lysates were collected and subjected to protein concentration detection using a BCA kit [42] . Equivalent protein concentrations of cell lysates were incubated with FITC-labelled AAN-TAT-Lipo-Dox at 37 °C for 2 h. The reaction mixture was then purified over a PD-10 column (GE), and resulting fractions were examined by spectral scanning. The cleavage efficiency of legumain was evaluated according to the respective fluorescence intensities of doxorubicin (OD=590 nm) and FITC (OD=520 nm) by spectral scanning analysis. Tumour growth and survival curves Eight-week-old female BALB/c mice were obtained from the Academy of Military Medical Sciences, Laboratory Animal Center (Peking, China). The mice were housed at the animal facilities of Nankai University with free access to food and water. The animal experiments were performed in accordance with institutional guidelines, and the study was approved by the ethics committee of Nankai University. An orthotopic mouse model of breast cancer was set up through the injection of 5 × 10 4 luciferase-expressing 4T1 cells suspended in 50 μl of PBS at the fourth mammary fat pad (left). Forty mice were randomly divided into five groups and received free doxorubicin or the equivalent amount of doxorubicin loaded into various carriers as indicated ( n =8): PBS, free doxorubicn, Lipo-Dox, TAT-Lipo-Dox, AAN-Lipo-Dox and AAN-TAT-Lipo-Dox. The mice were intravenously administrated with 1 nM free doxorubicin or the equivalent amount of doxorubicin loaded into the AAN-TAT-Lipo or other control nanoparticles or PBS every 3 days for five consecutive times from the 15th day after the injection of the tumour cells. The tumour volumes of the tumour-bearing mice were measured by a Xenogen IVIS2000 system (Caliper, Waltham, MA, USA) every 3 days from day 15 after the injection of the tumour cells. The mice were killed under anaesthesia when the tumours reached approximately 3,000 mm 3 in volume. The tumour tissue, kidney, liver and heart were isolated and placed onto frozen slides of 5 μm thickness. Data pertaining to the primary tumour diameter (>1.8 cm) and natural death were recorded as a survival curve. Biodistribution assay MDA-MB-231 human breast cancer, A549 human lung cancer and 4T1 mouse breast cancer models were established as follows. Stable luciferase-expressing MDA-MB-231 cells or stable luciferase -expressing A549 cells (1 × 10 6 ) were injected separately at the fourth mammary fat pad of NOD/SCID mice or intravenously administered via tail vein injection. Stable luciferase-expressing 4T1 cells (5 × 10 4 ) were orthotopically injected at the fourth mammary fat pad of BALB/c mice. When the tumour volume reached approximately 500 mm 3 , the mice were administered intravenously with DiR-labelled AAN-TAT-Lipo, AAN-Lipo or Lipo nanoparticles. The DiR signal was then measured 24 h after intravenous injection using a Xenogen IVIS2000 system (Caliper) with excitation and emission wavelengths of 750 and 780 nm, respectively. In the MDA-MB-231 human breast cancer mouse model, tumour-bearing mice were injected intravenously with free doxorubicin or an equivalent amount of doxorubicin loaded in the AAN-TAT-Lipo, AAN-Lipo or TAT-Lipo. After 24 h, mice were killed under anaesthesia, and their kidney, liver, heart and tumour tissues removed and prepared as homogenates. Doxorubicin was isolated from the tissues and its concentration in the tissue homogenates detected by a fluorescence plate reader at excitation and emission wavelengths of 480 and 590 nm, respectively. Statistical analyses Statistical analyses were performed using the GraphPad Software (La Jolla, CA, USA) and SigmaStat software (Jandel Scientific Software, San Rafael, CA, USA). Data were expressed as the mean values of at least three independent determinations±s.e.m., from experiments that had been performed in triplicate. Statistical significance was determined using the Student’s t -test, one-way analysis of variance, two-way analysis of variance or unpaired t -test. How to cite this article: Liu, Z. et al. Legumain protease-activated TAT-liposome cargo for targeting tumours and their microenvironment. Nat. Commun. 5:4280 doi: 10.1038/ncomms5280 (2014).